Time-resolved ultrafast photocurrents and terahertz generation in freely suspended graphene Graphene, a two-dimensional layer of carbon atoms, is a promising building block for a wide range of optoelectronic devices owing to its extraordinary electrical and optical properties, including the ability to absorb ~2% of incident light over a broad wavelength range. While the RC-limited bandwidth of graphene-based photodetectors can be estimated to be as large as 640 GHz, conventional electronic measurement techniques lack for analysing photocurrents at such frequencies. Here we report on time-resolved picosecond photocurrents in freely suspended graphene contacted by metal electrodes. At the graphene–metal interface, we demonstrate that built-in electric fields give rise to a photocurrent with a full-width-half-maximum of ~4 ps and that a photothermoelectric effect generates a current with a decay time of ~130 ps. Furthermore, we show that, in optically pumped graphene, electromagnetic radiation up to 1 THz is generated. Our results may prove essential to build graphene-based ultrafast photodetectors, photovoltaic cells and terahertz sources. The high charge-carrier mobility in graphene has spurred a tremendous interest in graphene-based high-speed electronic devices such as field-effect transistors and pn-junctions [1] , [2] . In combination with its excellent optical properties [3] , graphene further qualifies for optoelectronic applications [4] , [5] , [6] , [7] , [8] , [9] , [10] , [11] , [12] . Various graphene-based terahertz sources and detectors have been proposed, as the frequency of plasma waves, the gap of graphene nanoribbons, and the tunable bandgap in bilayer graphene lies in the terahertz range [3] , [13] , [14] , [15] , [16] . Whereas the RC-limited bandwidth of graphene-based photodetectors can be estimated to be as large as 640 GHz (ref. 12 ), common electronic apparatuses cannot resolve the underlying ultrafast charge-carrier dynamics because available equipment cannot produce electronic trigger signals and detect transients faster than tens of picoseconds. Here we introduce a pump-probe photocurrent spectroscopy to graphene-based devices to resolve their photo-electric response up to 1 THz (ref. 17 ). In our experiments, we demonstrate that terahertz radiation is generated in optically pumped graphene. The electromagnetic radiation is detected by a coplanar metal stripline, which acts as a highly sensitive near-field antenna and waveguide with a bandwidth of up to 1 THz. Our ultrafast experiments further clarify the optoelectronic mechanisms contributing to the photocurrent generation at graphene–metal interfaces. So far, this photocurrent has been extensively investigated by spatially resolved, but time-integrated photocurrent imaging techniques [3] , [4] , [5] , [6] . We verify that both built-in electric fields [4] , [7] , similar to those in semiconductor-metal interfaces [18] , and a photothermoelectric effect [6] , [19] give rise to the photocurrent at graphene–metal interfaces at different time scales. Our results open the possibility to design and fabricate graphene-based ultrafast photodetectors, photoswitches, photovoltaic cells, and terahertz sources [15] . Time-integrated and time-resolved photocurrent spectroscopy The investigated graphene sheets are fabricated as recently described [11] , [20] (Methods). We first measure the time-integrated, spatially resolved photocurrent I photo of the freely suspended graphene in the stripline circuit ( Fig. 1a ). At zero bias voltage V sd , we find two spatial extrema of I photo , each of which is in the vicinity of a metal electrode ( Fig. 1b,c ). The extrema are consistent with recent scanning photocurrent results [4] , [5] , [6] . They can be explained in terms of built-in electric fields or a photothermoelectric current at graphene–metal interfaces, as will be discussed below in detail. 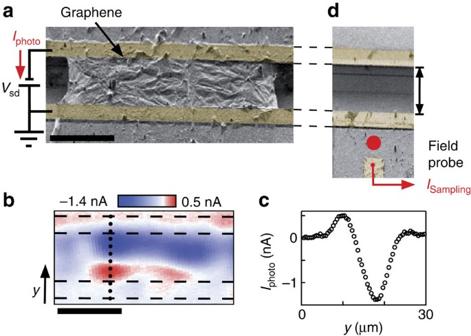Figure 1: Ultrafast photocurrent circuitry for graphene. (a) Freely suspended graphene is incorporated into a coplanar stripline circuit. A pump laser pulse focused onto the graphene-sheet generates the time-integrated photocurrentIphoto. Scale bar, 20 μm. (b) Spatially resolved scan ofIphoto. The position of the striplines is indicated with dashed lines. Scale bar, 20 μm. The experimental parameters areElaser=1.6 eV,Plaser=200 μW,Vsd=0 V, andTbath=300 K. (c) Single line-sweep ofIphotoalong the dotted line in (b). (d) The time-resolved photocurrent responseIsamplingis measured at the field probe, located ~0.3 mm away from the graphene. The probe laser pulse (red circle) triggers the read-out ofIsampling. Scale bar, 15 μm. Figure 1: Ultrafast photocurrent circuitry for graphene. ( a ) Freely suspended graphene is incorporated into a coplanar stripline circuit. A pump laser pulse focused onto the graphene-sheet generates the time-integrated photocurrent I photo . Scale bar, 20 μm. ( b ) Spatially resolved scan of I photo . The position of the striplines is indicated with dashed lines. Scale bar, 20 μm. The experimental parameters are E laser =1.6 eV, P laser =200 μW, V sd =0 V, and T bath =300 K. ( c ) Single line-sweep of I photo along the dotted line in ( b ). ( d ) The time-resolved photocurrent response I sampling is measured at the field probe, located ~0.3 mm away from the graphene. The probe laser pulse (red circle) triggers the read-out of I sampling . Scale bar, 15 μm. Full size image To investigate the temporal optoelectronic dynamics in graphene, we measure I sampling at the field probe as a function of the time delay t delay between the pump- and probe pulse ( Fig. 1d and Methods). 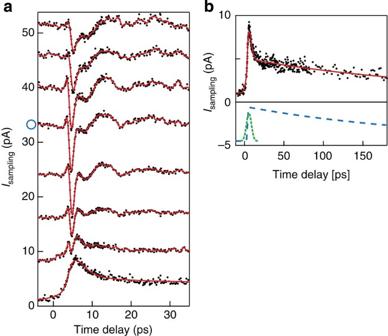Figure 2: Time-resolved photocurrents in graphene. (a)Isamplingfor excitation positions starting at the graphene–metal interface in steps of 2 μm (from bottom to top) along the dotted line inFigure 1b. Solid lines are guides to the eye. Data are offset for clarity. The experimental parameters areElaser=1.59 eV,Plaser=800 μW,Vsd=0 V, andTbath=300 K. (b) Lowest trace in (a) and its fitting function (solid line) fortdelayup to 180 ps. The individual components of the fitting function are offset for clarity and depicted as dashed and dotted lines. Figure 2a shows I sampling as a function of t delay for excitation positions starting at the graphene–metal interface in steps of 2 μm (from bottom to top along the dotted line in Fig. 1b ). The amplitude of the main peak of I sampling centred around 5 ps reverses sign from the lowest to the topmost trace. This finding is consistent with the spatial dependence of I photo ( Fig. 1b,c ), which indicates the direct correlation between the time-integrated I photo and the time-resolved I sampling (refs 18 , 21 ). Figure 2: Time-resolved photocurrents in graphene. ( a ) I sampling for excitation positions starting at the graphene–metal interface in steps of 2 μm (from bottom to top) along the dotted line in Figure 1b . Solid lines are guides to the eye. Data are offset for clarity. The experimental parameters are E laser =1.59 eV, P laser =800 μW, V sd =0 V, and T bath =300 K. ( b ) Lowest trace in ( a ) and its fitting function (solid line) for t delay up to 180 ps. The individual components of the fitting function are offset for clarity and depicted as dashed and dotted lines. Full size image Built-in electric field and photo-thermoelectric effect Generally, directly after an optical excitation of graphene, the photogenerated charge-carriers redistribute to decrease local potential differences. This displacement of the charge-carriers decreases the electric field E in the irradiated region. In turn, the optoelectronic response can be described by a transient displacement current density [22] , [23] This mechanism also holds for built-in electric fields and can produce displacement currents even with sub-picosecond duration [21] , [22] , [23] . The amplitude of the displacement current saturates if the electric field E is set to zero by the displacement of the optically excited charge-carriers. Figure 2b shows the trace of I sampling at the graphene–metal interface extended to t delay =180 ps (dots). The solid line is a fit with the sum of a Gaussian and an exponentially convoluted Gaussian, which are shown individually as dotted and dashed lines. 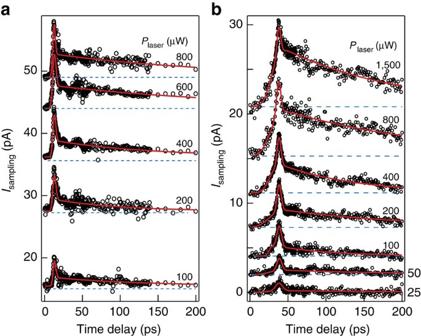Figure 3: Laser power dependence of the ultrafast photocurrent at the graphene–metal interface. Isamplingversustdelayas a function ofPlaserfor (a) sample #1 and (b) sample #2 at room temperature. Lines are fits to the data. The data offset level is indicated with dashed lines. The experimental parameters areElaser=1.59 eV,Vsd=0 V andTbath=300 K. In Figure 3a,b , we depict data of the optoelectronic response of two samples #1 and #2 measured at the graphene–metal interface as a function of the laser power. Sample #1 is the graphene device, which is further characterized in Figures 1 and 2 . The data in Figure 3 are taken down to a power level where the experimental noise dominates the signal. With both samples, we detect a fast optoelectronic signal in combination with a slowly decaying current component. For sample #2 ( Fig. 3b ), the onset of I sampling at short t delay is less steep compared with the data on sample #1 ( Fig. 3a ). We interpret this to stem from a slightly enhanced dispersion and attenuation for sample #2, because, for this sample, the detected electromagnetic pulses propagate along a longer graphene-covered part of the stripline [24] . We present the integrated area of the fast first peak for sample #1 (#2) as green symbols in Fig. 4a (b). Most importantly, the area of the first peak increases as a function of P laser and then, for P laser ≥ 200 μW, it saturates at a constant value. 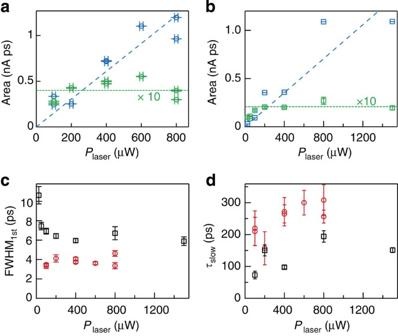Figure 4: Fit parameters forIsamplingversusPlaserat the graphene–metal interface. Area of the individual components of the fitting function for (a) sample #1 and (b) sample #2. Green symbols represent the area of the fast first peak. The blue symbols stand for the area of the exponentially convoluted slow Gaussian peak. Dashed and dotted lines are linear fits. (c) FWHM of the first peak as a function ofPlaserfor sample #1 (red) and sample #2 (black). (d)τslowfor both samples as a function ofPlaserfor sample #1 (red) and sample #2 (black). Error bars reflect the estimated standard deviation of the fit coefficients. Figure 4c shows the full-width-half-maximum (FWHM) of the first peak for both samples #1 and #2. In both cases, the FWHM stays rather constant throughout the examined laser power range with a mean average of 4.3±0.1 ps. The slightly increased fitted values for sample #2 at small laser powers can be explained by the impact of the noise. Most importantly, there is a range of P laser where the FWHM and the area of the first fast peak are constant within the experimental error for both samples #1 and #2. Taking all the above arguments together, we interpret the fast peak with a FWHM ~4 ps to stem from the ultrafast screening of the electric fields at the graphene–metal interface by the displacement of the photogenerated charge-carriers. Consistently, its FWHM of (4.3±0.1) ps is comparable to values found in carbon nanotubes [18] (~2.1 ps) and low temperature grown (LT)-gallium arsenide [21] (~1.5 ps), all measured in similar stripline circuits. We conclude that a displacement current due to built-in electric fields at the graphene–metal interface is generating this ultrafast photoresponse. Furthermore, we note that the fast peak is not related to a thermoelectric effect induced by electrons, because such an effect cannot explain the saturation of the peak area for larger values of P laser . Figure 3: Laser power dependence of the ultrafast photocurrent at the graphene–metal interface. I sampling versus t delay as a function of P laser for ( a ) sample #1 and ( b ) sample #2 at room temperature. Lines are fits to the data. The data offset level is indicated with dashed lines. The experimental parameters are E laser =1.59 eV, V sd =0 V and T bath =300 K. Full size image Figure 4: Fit parameters for I sampling versus P laser at the graphene–metal interface. Area of the individual components of the fitting function for ( a ) sample #1 and ( b ) sample #2. Green symbols represent the area of the fast first peak. The blue symbols stand for the area of the exponentially convoluted slow Gaussian peak. Dashed and dotted lines are linear fits. ( c ) FWHM of the first peak as a function of P laser for sample #1 (red) and sample #2 (black). ( d ) τ slow for both samples as a function of P laser for sample #1 (red) and sample #2 (black). Error bars reflect the estimated standard deviation of the fit coefficients. Full size image The area of the exponentially convoluted slow Gaussian peak, however, increases linearly with P laser for the examined range of laser power (blue symbols in Fig. 4a,b ). This suggests that the exponentially convoluted Gaussian is associated with a thermoelectric effect, because the thermovoltage U thermo can be described as, where Δ T is the optically induced temperature difference and S graphene and S stripline are the Seebeck coefficients of graphene and the metal stripline [6] . For small P laser , one expects that Δ T and, therefore, U thermo linearly depend on P laser . On the basis of the linear power dependence in Figure 4a,b , we interpret the slowly decaying photoresponse contribution in Figures 2 and 3 to be caused by a short-time temperature difference ΔT between the graphene and the metal. The interpretation is further corroborated by the fact that τ slow is rather constant for the examined range of P laser within the experimental error ( Fig. 4d ). The mean value of τ slow =130±10 ps (for both samples) suggests that Δ T is dominated by heat diffusion rates along the metal stripline [25] . Photocurrent oscillations in freely suspended graphene For an optical excitation in the middle of the freely suspended graphene, we detect strong oscillations of I sampling that start at t delay ~5 ps ( Fig. 2a ). The oscillatory amplitude increases towards the centre of the graphene. We investigate the oscillations by performing a fast-Fourier-transformation (FFT) ( Fig. 5a ) of the I sampling trace indicated with an open circle in Figure 2a . Most prominently, we find amplitudes at frequencies up to 0.8 THz. The oscillatory behaviour of I sampling does not have a counterpart in the time-integrated I photo , which decreases from the contacts towards the middle of the graphene ( Fig. 1c ). At the graphene–metal interfaces (for example, lowest trace in Fig. 2a ), the photo-thermoelectric effect and built-in electric fields dominate the optoelectronic response. Therefore, the fast oscillations of I sampling are generic to the freely suspended graphene sections. 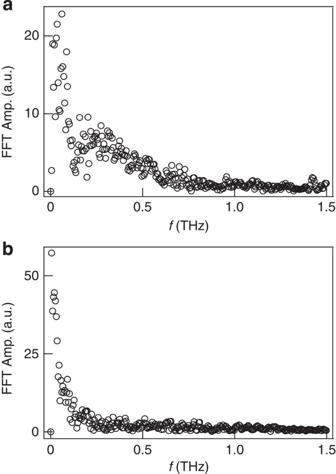Figure 5: Frequency analyis of ultrafast photocurrents in graphene. (a) FFT ofIsamplingfor excitation in the centre of the freely suspended graphene (fourth trace from the top inFig. 2a). (b) FFT ofIsamplingfor the excitation position close to the metal contact (lowest trace inFig. 2a). For comparison, Figure 5b shows a FFT of I sampling measured at the graphene–metal interface (lowest trace in Fig. 2a ). Figure 5: Frequency analyis of ultrafast photocurrents in graphene. ( a ) FFT of I sampling for excitation in the centre of the freely suspended graphene (fourth trace from the top in Fig. 2a ). ( b ) FFT of I sampling for the excitation position close to the metal contact (lowest trace in Fig. 2a ). 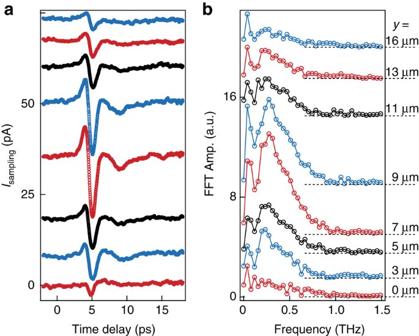Figure 6: Terahertz response of graphene. (a) Time-resolvedIsamplingatTbath=77 K for excitation positions starting at the graphene–metal interface along the dotted line inFig. 1b. Data are offset for clarity. The experimental parameters areElaser=1.59 eV,Plaser=800 μW, andVsd=0 V. (b) Corresponding fast-Fourier-transformation of interpolatedIsamplingas displayed in (a). The positionyrefers to the dotted line inFigure 1b. The data offset level is indicated with dashed lines. Full size image In Figure 6a , we show I sampling measured at a bath temperature of T bath =77 K, for excitation positions along the dotted line in Figure 1b . In a first approximation, S graphene linearly depends on the temperature [19] , [26] . Therefore, we expect a decrease of the thermoelectrically induced ultrafast photocurrent to about 1/4 of its room-temperature value when lowering T bath down to 77 K. Indeed, at the graphene–metal interface, the slow-decaying signal of I sampling is suppressed ( Fig. 6a ). In the middle of the freely suspended graphene, however, fast oscillations of I sampling again occur for t delay ≥5 ps. The FFT yields amplitudes for frequencies up to 1 THz ( Fig. 6b ). Figure 6: Terahertz response of graphene. ( a ) Time-resolved I sampling at T bath =77 K for excitation positions starting at the graphene–metal interface along the dotted line in Fig. 1b . Data are offset for clarity. The experimental parameters are E laser =1.59 eV, P laser =800 μW, and V sd =0 V. ( b ) Corresponding fast-Fourier-transformation of interpolated I sampling as displayed in ( a ). The position y refers to the dotted line in Figure 1b . The data offset level is indicated with dashed lines. 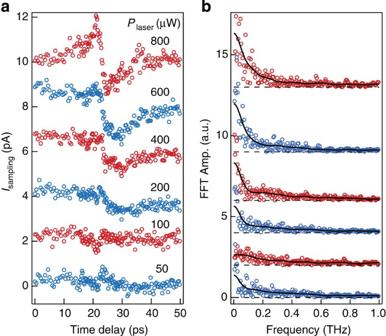Figure 7: Power dependence ofIsamplingat the centre of the graphene. (a) Fast oscillatory part ofIsamplingat the centre of the graphene as a function oftdelayfor differentPlaser. (b) Corresponding fast-Fourier-transformation of interpolatedIsamplingas displayed in (a). Interpolating lines act as guide to the eye. The data offset level is indicated with dashed horizontal lines. Full size image In Figure 7a , we depict data of the optoelectronic response at the centre of the graphene sample #1 as a function of the laser power. The data are taken after the sample was temperature-cycled several times in the course of the optoelectronic experiments. It exhibits a worse signal to noise ratio as compared with the data presented in Figure 2 , which were taken directly after the graphene was transferred onto its stripline circuit. Generally, the data in Figure 7a are taken down to a power level where the experimental noise dominates the signal. Again, we detect a fast oscillatory signal of I sampling . Figure 7b depicts the corresponding amplitude of a FFT of the data. Within the experimental error, the FFT-spectra shift to higher frequencies for increasing P laser . This can be directly seen also in the raw data in Figure 7a . For the highest P laser , the signal becomes 'steeper'. Figure 7: Power dependence of I sampling at the centre of the graphene. ( a ) Fast oscillatory part of I sampling at the centre of the graphene as a function of t delay for different P laser . ( b ) Corresponding fast-Fourier-transformation of interpolated I sampling as displayed in ( a ). Interpolating lines act as guide to the eye. The data offset level is indicated with dashed horizontal lines. 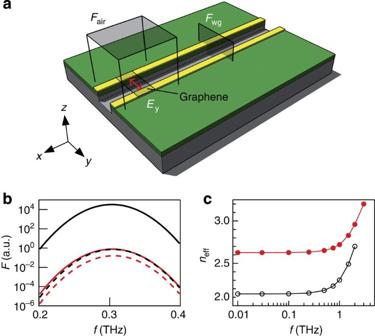Figure 8: Finite-difference-time-domain and finite-element-method simulation. (a) Sketch of the FDTD simulation geometry. Metal strips are indicated in yellow, the substrate in green and grey.FairandFwgindicate rectangular areas for calculating the passing field flux above and in the stripline circuit, respectively. (b) Field fluxFwg(solid black line) and field fluxFair(dashed black line) as a function of frequencyfin the FDTD simulation. The centre frequency isf=0.3 THz with a frequency width Δf=0.2 THz. Field fluxes for a simulation geometry without metal strips and trench are strongly reduced (Fwgred line,Fairdashed red line). (c) Finite-element-method simulation of the effective index of diffractionneffas a function of frequencyfwith (black circles) and without (full red circles) a trench. Solid lines are guides to the eye. Full size image Numerical stripline investigations Figure 8a shows a sketch of the graphene incorporated into a coplanar stripline circuit. The metal electrodes are depicted in yellow, the LT–GaAs in green. The metal striplines act as a near-field antenna, greatly enhancing the out-coupling of electromagnetic fields in the direction of the stripline. A finite-difference time-domain simulation (FDTD) is carried out to compare the radiation coupled into the metal stripline with the radiation emitted perpendicular to the sample surface, using a freely available software package [27] . In our simulation, a Gaussian electric field source E y (centre-frequency f =0.3 THz and width 0.2 THz) polarized along the y axis is placed inside the stripline ( Fig. 8a ). A 20-μm×20-μm window lying in the y – z plane is placed at a distance of 130 μm from the source E y centred with the stripline. The field flux F wg coupled into the stripline is measured in this window. The field flux F air radiated perpendicular to the sample surface is measured in a window of the same size, placed at the same distance of 130 μm directly above the field source E y . Figure 8b shows the field fluxes F as a function of frequency f . The field flux F wg (solid black line) at the centre-frequency is about a factor of 45,600 enhanced when compared with the field flux F air above the surface (dashed black line). We would like to mention here that increasing the propagation distance both along the stripline and perpendicular to the surface further increases the enhancement factor. Although the electric field E of a spherical wave decreases with the distance r with | E |~1/ r , it has been shown that the electromagnetic field of picosecond pulses can propagate along striplines for several millimeters with experiencing a small loss of ~35% (ref. 28 ). We therefore conclude that measuring the terahertz wave generation on-chip in a stripline circuit is several orders of magnitude more sensitive than measuring in a free-space set-up. However, omitting the trench and the metal stripline greatly reduces the field flux F wg (solid red line), and in turn, the enhancement factor is reduced to 150 when compared with the field flux F air above the surface (dashed red line). Figure 8: Finite-difference-time-domain and finite-element-method simulation. ( a ) Sketch of the FDTD simulation geometry. Metal strips are indicated in yellow, the substrate in green and grey. F air and F wg indicate rectangular areas for calculating the passing field flux above and in the stripline circuit, respectively. ( b ) Field flux F wg (solid black line) and field flux F air (dashed black line) as a function of frequency f in the FDTD simulation. The centre frequency is f =0.3 THz with a frequency width Δ f =0.2 THz. Field fluxes for a simulation geometry without metal strips and trench are strongly reduced ( F wg red line, F air dashed red line). ( c ) Finite-element-method simulation of the effective index of diffraction n eff as a function of frequency f with (black circles) and without (full red circles) a trench. Solid lines are guides to the eye. Full size image Generally, the spectral response of our measurements is limited to below 1 THz by the bandwidth of our detection scheme [29] . Figure 8c shows a finite-element-simulation of the odd-mode effective index of refraction n eff as a function of frequency for a 5/15/5 μm stripline circuit fabricated on a GaAs substrate. The effective index of refraction n eff is significantly reduced when a 12-μm deep trench located between the metal strips is considered (open circles), compared with a simulation without a trench (red circles). For the trench geometry, we estimate the effective index to be n eff =2.2±0.1 for frequencies below 1 THz. The dispersion for both geometries sets in at about 1 THz, thereby limiting our detection sensitivity to below 1 THz. For striplines without an etched trench and without graphene, the bandwidth of our detection scheme is also experimentally determined to be about 1 THz ( Supplementary Fig. S1 ). Generally, photoexcited charge-carriers in graphene can very efficiently relax by the emission of optical phonons with a subsequent interband recombination or via plasmon emission on a sub-picosecond timescale [15] , [16] , [30] , [31] , [32] . Our detection scheme is only sensitive to coherent electromagnetic radiation with constant phase with respect to each pulsed laser excitation. We therefore do not expect incoherent interband-recombination processes to contribute to the oscillations of I sampling . In the case of stimulated emission, the phase would be random with respect to each pulsed laser excitation. Indications for the creation of an electron-hole plasma in graphene after photoexcitation have recently been reported [33] , [34] . The frequency of electron-hole plasmons are predicted to be in the terahertz regime [15] . We therefore interpret the fact that we detect an oscillatory signal I sampling to be an indication of an electron-hole plasma in the graphene, which is AC-coupled to the striplines. We point out that our stripline detection scheme is a factor of 10 4 –10 5 more sensitive than a far-field detection of electromagnetic radiation in the tested frequency range ( Fig. 8b ). We further note that M. Freitag et al . recently reported on the thermal emission from graphene, which was heated by an electric current to a temperature of several tens to hundreds of kelvin [35] . A thermal emission, however, cannot explain a coherent emission of photons. Therefore, we infer that thermal emission of the photoexcited graphene is only of minor importance to describe our results. In conventional semiconductors, a symmetry-breaking due to (intrinsic) electric fields and/or different effective electron and hole diffusivities can lead to a preferential initial phase of the resulting terahertz plasma oscillations [36] ( Supplementary Fig. S2 ). In pristine graphene, however, both intrinsic fields [4] and a difference between effective charge carrier masses are absent [1] , [2] . To explain our experiments, we interpret the required symmetry breaking to stem from the overall nonuniformity of the samples or from an ultrafast interaction between the few (1–3) individual layers of graphene. As has been reported for graphite [37] , collective carrier and phonon dynamics can be induced by plasmons ~180 fs after an ultrafast optical near-infrared excitation. In our experiment, the centre frequency of the high-frequency components at ~300 GHz does not shift strongly with excitation position ( Fig. 6b ). However, it shifts to higher frequencies with increasing excitation laser power ( Fig. 7 ). The latter finding corroborates our interpretation that a plasmonic excitation generates the terahertz radiation. We further note that the low-frequency components (<100 GHz) in the FFT spectrum in Figure 6b possibly originate from reflections of the electromagnetic pulse at irregularities of the metal stripline. For instance, a frequency of translates into a distance along the stripline of d ~ t travel · c 0 / n eff =10 ps· c 0 /(2.2±0.1)~(1.36±0.06) mm (see Fig. 8c for n eff ). However, by using optical microscopy, we could not identify an apparent imperfection of the stripline circuits explaining the low-frequency components. Another possibility is given by reflections of the terahertz radiation emitted from the graphene at the boundaries of the GaAs-wafer. A terahertz pulse, which is reabsorbed at the position of the field probe, would be expected at earliest at a time delay of t =2· w · n GaAs / c 0 ~8.4 ps and later, with w =350 μm the height of the substrate and n GaAs the diffraction index of GaAs. Therefore, we tentatively attribute the variation of the low-frequency components in Figure 6b by such reflections. Generally, we only subtract an offset level from the original finite-size data before the fast-Fourier transformation. In respect of electronically contacting graphene, we remark that the terahertz signal in Figure 6 decreases towards the metal contacts. In our interpretation, the photothermoelectric and displacement currents contribute to I sampling at the graphene–metal interface. At room temperature, all processes can be concurrently resolved at specific excitation positions, for example the second trace from the bottom in Figure 2a . At 77 K, however, we cannot resolve the photothermoelectric and displacement currents at the metal–graphene interface because of a dominating terahertz response. To conclude, we spatially resolve picosecond photocurrents in freely suspended graphene contacted by metal striplines. We identify both built-in electric fields and the photothermoelectric effect to contribute to the photocurrent generation at graphene–metal interfaces. In addition, optical pumping of the freely suspended graphene gives rise to strong photocurrent oscillations in the time-domain. We interpret these oscillations with FFT-amplitudes up to 1 THz to originate from terahertz radiation emitted from an electron-hole plasma in the optically pumped graphene. Fabrication of the suspended graphene The studied graphene samples were directly synthesized on copper (Cu) foil using liquid precursor hexane in a chemical vapour deposition system [20] . After growth, a thin poly-methyl-meth-acrylate (PMMA) film was deposited on the graphene/Cu substrate as supporting layer for the graphene transfer. The underlying Cu substrate was then dissolved in dilute HNO 3 and washed several times in deionized water. The floating graphene/PMMA film was controllably transferred onto a pre-processed GaAs substrate, such that the graphene spans two electrodes of a gold stripline. The sample was immersed into acetone solvent to remove PMMA, and then dried in critical point dryer to avoid the damage of the freely suspended graphene by liquid surface tension. In this procedure, we obtain one to three graphene layers ( Supplementary Fig. S3 ). Precursor-assisted scanning-electron-beam deposition of platinum onto the graphene covering the stripline is used to lower the contact resistance of sample #1. Sample #2 comprises a freely suspended graphene layer as sample #1. However, this layer is not further contacted by electron-beam-induced Pt deposition at the stripline electrodes. The freely suspended graphene and the two electrodes of the stripline form a two-terminal circuit driven by a bias voltage V sd ( Fig. 1a ). The two-terminal resistance of the graphene devices is in the order of 1.7 kΩ at 300 K and 0.9 kΩ at 77 K. Design of the stripline circuit The LT–GaAs is grown by molecular beam epitaxy on a GaAs substrate. In growth order, the layers are: 350 μm GaAs, 400 nm Al 0.3 Ga 0.7 As, and 2 μm of LT–GaAs. After growth, the heterostructure is annealed at 600 °C within an O 2 -rich environment. 5/15/5 μm coplanar striplines are fabricated by optical lithography: the two Au electrodes of the stripline are 5-μm wide, 200-nm high, and they have a separation of 15 μm. Inductively coupled plasma reactive-ion etching is used to define a 12-μm deep trench in between the two electrodes throughout the whole stripline, using 50 nm Ni as an etch mask. Time-resolved photocurrent measurements The suspended graphene in the stripline circuit is optically excited by a pump-pulse with ~160-fs pulse length generated by a titanium:sapphire laser with a photon energy of E laser =1.59 eV. After excitation, an electromagnetic pulse starts to travel along the stripline [17] , [18] , [21] . A field probe senses the transient electric field of the travelling pulse ( Fig. 1d ). Here we utilize an Auston-switch based on the LT–GaAs substrate. This Auston-switch at the field probe is short-circuit by the probe laser-pulse for the duration of the lifetime ≤1 ps of the photo-generated charge-carriers in the LT–GaAs. The transient electric field located at the field probe during this time-period drives the current I sampling into the field probe. The time-delay t delay between the pump- and the probe pulse is controlled by a delay stage. Measuring the current I sampling at the field probe as a function of t delay yields information on the optoelectronic response of the graphene with a picosecond time resolution [18] . The time an electromagnetic pulse travels from the graphene to the field probe can be estimated via t travel = d · n eff / c 0 =0.3 mm·(2.2±0.1)/ c 0 ~(2.2±0.3) ps (see Fig. 8c for n eff ). The striplines have a total length exceeding 48 mm. Thus, reflections at the end of the striplines are expected for t delay ≥ 350 ps. The amplitude of the reflections is strongly reduced due to damping and radiation losses. Therefore, no reflections overlap with the electromagnetic signal coming directly from the graphene in our data. The position of the pump-spot y perpendicular to the stripline is set by a scanning mirror with a resulting spatial resolution of ~100 nm, while the position of the probe-spot is kept constant throughout the experiments. All room-temperature measurements of I sampling were carried out utilizing an optical chopper system, a current-voltage-converter connected to the field probe, and a lock-in amplifier. The measurements at 77 K were carried out with a retroreflector oscillating at 20 Hz and an oscilloscope, which averaged 128 times for each excitation position. The spot size of the pump laser is (2.0±0.2) μm. The laser power of the pump (probe) pulse is chosen to be in the range of 100–800 μW (50–120 mW). The presented results depend linearly on the laser power of the probe pulse. All data are taken in vacuum (~10 −5 mbar) to prevent the effect of photodesorption of oxygen on the surface of the graphene. Supplementary information accompanies this paper at http://www.nature.com/naturecommunications . How to cite this article: Prechtel L. Time-resolved ultrafast photocurrents and terahertz generation in freely suspended graphene. Nat. Commun. 3:646 doi: 10.1038/ncomms1656 (2012).